Engineering biosynthetic excitable tissues from unexcitable cells for electrophysiological and cell therapy studies Patch-clamp recordings in single-cell expression systems have been traditionally used to study the function of ion channels. However, this experimental setting does not enable assessment of tissue-level function such as action potential (AP) conduction. Here we introduce a biosynthetic system that permits studies of both channel activity in single cells and electrical conduction in multicellular networks. We convert unexcitable somatic cells into an autonomous source of electrically excitable and conducting cells by stably expressing only three membrane channels. The specific roles that these expressed channels have on AP shape and conduction are revealed by different pharmacological and pacing protocols. Furthermore, we demonstrate that biosynthetic excitable cells and tissues can repair large conduction defects within primary 2- and 3-dimensional cardiac cell cultures. This approach enables novel studies of ion channel function in a reproducible tissue-level setting and may stimulate the development of new cell-based therapies for excitable tissue repair. All cells express ion channels in their membranes, but cells with a significantly polarized membrane that can undergo a transient all-or-none membrane depolarization (action potential, AP) are classified as 'excitable cells' [1] . The coordinated function of ion channels in excitable cells governs the generation and propagation of APs, which enable fundamental life processes such as the rapid transfer of information in nerves [2] and the synchronized pumping of the heart [3] . For this reason, genetic or acquired alterations in ion channel function or irreversible loss of excitable cells through injury or disease (for example, stroke or heart attack) are often life threatening [4] , [5] . Numerous ion channels (wild type (wt) or mutated) have been studied in single-cell heterologous expression systems to investigate channel structure–function relationships and link specific channel mutations found in patients to associated diseases, such as cardiac arrhythmias or epilepsy [6] . Typically, the potential implications of these single-cell studies for the observed tissue- or organ-level function are only speculated, often through the use of tissue-specific computational models [7] , [8] . Similarly, experimental studies of AP conduction in primary excitable tissues and cell cultures are often limited by low reproducibility, heterogeneous structure and function, a diverse and often unknown complement of endogenous channels, and the non-specific action of applied pharmaceuticals. We therefore set out to develop and validate a simplified, well-defined and reproducible excitable tissue system that would enable direct quantitative studies of the roles that specific ion channels have in AP conduction. Extensive electrophysiological research over the last century [1] , [9] has revealed that the initiation, shape and transfer of APs in excitable cells are regulated by an extraordinarily diverse set of ion channels, pumps and exchangers. Yet, the classic Hodgkin and Huxley bioelectric model of a giant squid axon [10] and other simplified models of biological excitable media [11] , [12] suggest that only a few membrane channels are sufficient to sustain cellular excitability and AP conduction. On the basis of these theoretical concepts, we hypothesized that a small number of targeted genetic manipulations could transform unexcitable somatic cells into an electrically active tissue capable of generating and propagating APs. In this study, we selected a minimum set of channel genes that, upon stable expression in unexcitable cells, would yield significant hyperpolarization of membrane potential, electrical induction of an all-or-none AP response and robust intercellular electrical coupling to support uniform and fast AP conduction over arbitrarily long distances. We designed experiments to thoroughly characterize the electrophysiological properties of these genetically engineered cells including pharmacological manipulations to establish the roles of each of the expressed channels in membrane excitability and impulse conduction. Furthermore, we explored whether these cells could be used to generate biosynthetic excitable tissues with the ability to restore electrical conduction within large cm-sized gaps in primary excitable cell cultures. Experimental approach to engineering excitable cells We tested the hypothesis that human unexcitable somatic cells can be genetically engineered to form an autonomous source of electrically excitable and conducting cells through the stable expression of three genes encoding: the inward-rectifier potassium channel (Kir2.1 or IRK1, gene KCNJ2 ) [13] , the pore-forming α-subunit of the fast voltage-gated cardiac sodium channel (Na v 1.5 or hH1, gene SCN5A ) [14] and the connexin-43 gap junction (Cx43, gene GJA1 ) [15] . These three channels have critical roles in the generation and propagation of electrical activity in the mammalian heart [16] , [17] . To facilitate the visual identification and monoclonal selection of stable cell lines, we constructed three bicistronic plasmids designed to express each channel (Kir2.1, Na v 1.5 or Cx43) with a unique fluorescent reporter [18] (mCherry, green fluorescent protein (GFP) or mOrange, respectively) and the puromycin resistance ( PacR ) gene ( Supplementary Fig. S1 ). The human embryonic kidney 293 (HEK-293) cell line was utilized as a proof-of-concept unexcitable somatic cell source based on its low levels of endogenous membrane currents (for example, outwardly rectifying potassium currents [19] ), uniform shape and growth, and extensive use as a heterologous expression system for studies of ion channel function [20] . Like most unexcitable cells, wt HEK-293 cells ( Fig. 1a ) exhibited a relatively depolarized resting membrane potential (RMP) of −24.4±0.8 mV (±s.e.m. ; n =10 cells; Fig. 1b ). In contrast, the RMP of excitable cells is highly negative due to the action of constitutively open and/or inwardly rectifying potassium channels such as Kir2.1 (ref. 21 ). 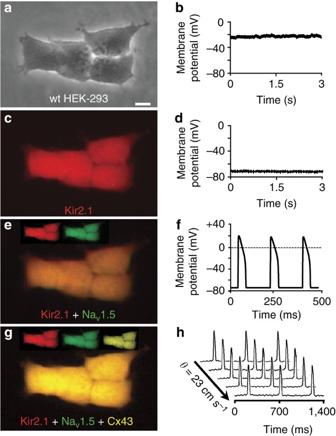Figure 1: Stable coexpression of three genes confers impulse conduction in unexcitable cells. wt HEK-293 cells (a), like most unexcitable cells, have a relatively depolarized resting potential (b). Scale bar, 10 μm. Stable expression of Kir2.1-IRES-mCherry (c) introduces inward-rectifier potassium current in the cell yielding membrane hyperpolarization (d). Coexpression of Nav1.5–IRES–GFP (e) introduces fast sodium current that allows firing of regenerative APs on stimulation (f). The additional expression of Cx43–IRES–mOrange (g) enhances cell–cell coupling and enables fast and uniform AP propagation (h) in multicellular tissues.θ, Velocity of AP propagation. Figure 1: Stable coexpression of three genes confers impulse conduction in unexcitable cells. wt HEK-293 cells ( a ), like most unexcitable cells, have a relatively depolarized resting potential ( b ). Scale bar, 10 μm. Stable expression of Kir2.1-IRES-mCherry ( c ) introduces inward-rectifier potassium current in the cell yielding membrane hyperpolarization ( d ). Coexpression of Na v 1.5–IRES–GFP ( e ) introduces fast sodium current that allows firing of regenerative APs on stimulation ( f ). The additional expression of Cx43–IRES–mOrange ( g ) enhances cell–cell coupling and enables fast and uniform AP propagation ( h ) in multicellular tissues. θ , Velocity of AP propagation. Full size image I K1 and I Na expression enables AP generation To induce significant membrane hyperpolarization in the wt HEK-293 cells, we stably transfected them with a plasmid encoding Kir2.1–IRES–mCherry and derived 'Kir2.1 HEK-293' monoclonal lines from cells that displayed bright mCherry fluorescence ( Fig. 1c ). These stable cell lines exhibited robust barium-sensitive inward-rectifier potassium current, I K1 ( Supplementary Fig. S2 and Fig. 2a,b ), and hyperpolarized RMP values ( Fig. 2c ) similar to those of primary excitable cells [1] . A hyperpolarized RMP is required for cellular excitability, as it allows a sufficient number of voltage-gated sodium channels to open on membrane depolarization and initiate a regenerative AP [16] , [17] . In addition, a hyperpolarized RMP, as a natural state of excitable cells, has been shown to distinctly affect the expression level and kinetics of ion channels [22] , [23] . 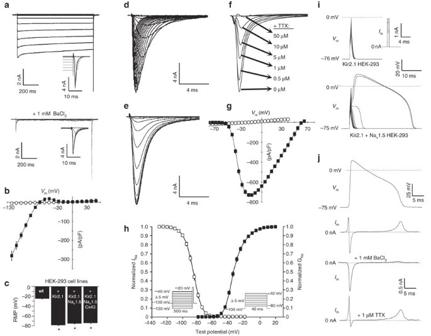Figure 2: Stable expression of Kir2. 1 and Nav1.5 yields membrane excitability in HEK-293 cells. (a) Kir2.1+Nav1.5 HEK-293 cells exhibited BaCl2-sensitiveIK1. Activation ofINaalso occurred at the end of severalIK1test pulses (insets). (b) Steady-stateIK1–V curves obtained from Kir2.1+Nav1.5 (black squares;n=9) and wt (white circles;n=6) HEK-293 cells. (c) Expression ofIK1yielded significant hyperpolarization of RMP (n=10–27). Representative recordings ofINaactivation (d), inactivation (e) and TTX block (f) in Kir2.1+Nav1.5 HEK-293 cells. (g) PeakINa–V curves obtained from Kir2.1+Nav1.5 (black squares;n=6) and wt HEK-293 (white circles;n=6) cells. (h) Voltage dependence ofINasteady-state activation (black squares;n=6) and inactivation (white squares;n=6). (i) Current pulses (inset) induced an all-or-none AP response in Kir2.1+Nav1.5 but not in Kir2.1 HEK-293 cells. (j) AP-clamp recordings in Kir2.1+Nav1.5 HEK-293 cells revealed the individual contributions ofINaandIK1to the AP. Error bars denote mean±s.e.m.; *P<0.001;#P<0.01; and ^P<0.05. All recordings shown were made using the same monoclonal Kir2.1+Nav1.5 HEK-293 cell line. Figure 2: Stable expression of Kir2. 1 and Na v 1.5 yields membrane excitability in HEK-293 cells. ( a ) Kir2.1+Na v 1.5 HEK-293 cells exhibited BaCl 2 -sensitive I K1 . Activation of I Na also occurred at the end of several I K1 test pulses (insets). ( b ) Steady-state I K1 –V curves obtained from Kir2.1+Na v 1.5 (black squares; n =9) and wt (white circles; n =6) HEK-293 cells. ( c ) Expression of I K1 yielded significant hyperpolarization of RMP ( n =10–27). Representative recordings of I Na activation ( d ), inactivation ( e ) and TTX block ( f ) in Kir2.1+Na v 1.5 HEK-293 cells. ( g ) Peak I Na –V curves obtained from Kir2.1+Na v 1.5 (black squares; n =6) and wt HEK-293 (white circles; n =6) cells. ( h ) Voltage dependence of I Na steady-state activation (black squares; n =6) and inactivation (white squares; n =6). ( i ) Current pulses (inset) induced an all-or-none AP response in Kir2.1+Na v 1.5 but not in Kir2.1 HEK-293 cells. ( j ) AP-clamp recordings in Kir2.1+Na v 1.5 HEK-293 cells revealed the individual contributions of I Na and I K1 to the AP. Error bars denote mean±s.e.m. ; * P <0.001; # P <0.01; and ^ P <0.05. All recordings shown were made using the same monoclonal Kir2.1+Na v 1.5 HEK-293 cell line. Full size image To generate electrically excitable cells, we introduced a voltage-gated sodium channel, Na v 1.5, into a monoclonal Kir2.1 HEK-293 cell line by transfection of a plasmid encoding Na v 1.5–IRES–GFP ( Supplementary Fig. S1b ). We then selected cells with strong GFP expression to derive monoclonal 'Kir2.1+Na v 1.5 HEK-293' cells ( Fig. 1e ) that generated large, fast-inactivating sodium current, I Na ( Fig. 2d-g ). This current showed cardiac-specific sensitivity to block by tetrodotoxin (TTX; Fig. 2f ) and characteristic voltage-dependent steady-state activation and inactivation properties [14] ( Fig. 2h ). Importantly, much like primary excitable cells, the HEK-293 cells genetically engineered to stably express both I K1 and I Na developed membrane excitability, wherein on reaching an excitation threshold by current injection, they reproducibly fired an 'all-or-none' AP ( Figs 1f and 2i ). To dissect the contributions of I K1 and I Na to an AP time course in these cells, we utilized the AP-clamp technique [24] ( Fig. 2j ). As expected from the I K1 current–voltage relationship ( Fig. 2b ), outward potassium current activated above the resting potential during the AP upstroke in an attempt to maintain membrane hyperpolarization and also during AP plateau negative to −25 mV to bring the cell back to rest. Inward I Na activated only during the AP upstroke, followed by rapid inactivation ( Fig. 2j ). Cx43 expression enables rapid AP propagation We further tested whether the excitable Kir2.1+Na v 1.5 HEK-293 cells can support active electrical conduction when cultured in confluent two-dimensional (2D) cell networks. Optical mapping of transmembrane voltage in these cultures, however, revealed either uncoordinated aperiodic electrical activity caused by slowly moving and colliding excitation waves [25] or slow AP conduction (5.6±0.2 cm s −1 (±s.e.m. ; n =4); Fig. 3a,b ). This slow or unorganized AP propagation in the Kir2.1+Na v 1.5 HEK-293 cells was supported by weak endogenous cell coupling ( Supplementary Fig. S3a,b ) that likely originated from expression of connexin-45 (refs 26 , 27 ) rather than connexin-43 gap junctions ( Fig. 3c , inset) [27] , [28] . Therefore, to enable rapid and uniform AP propagation in the Kir2.1+Na v 1.5 HEK-293 cells, we stably transfected the monoclonal line characterized in Figure 2 with a plasmid encoding Cx43–IRES–mOrange ( Supplementary Fig. S1c ). 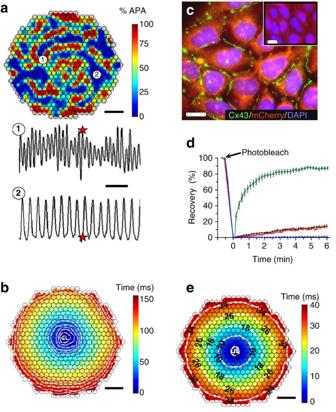Figure 3: Stable overexpression of Cx43 in Kir2. 1+Nav1.5 HEK-293 cells yields enhanced intercellular coupling and permits rapid AP propagation. (a) At the start of recording, confluent isotropic 2D networks (monolayers) of monoclonal Kir2.1+Nav1.5 cells usually exhibited high-frequency unorganized electrical activity caused by numerous, slowly moving, splitting and colliding waves. Shown is one instant of optically recorded transmembrane voltage. Colour bar indicates percent AP amplitude (% APA). Different sites in the monolayer (for example, 1 and 2) activated at different rates (bottom panel), demonstrating the lack of spatial synchrony in activation. Red stars denote the time at which the transmembrane voltage frame (top panel) was taken. Scale bars indicate 3 mm (top panel) and 250 ms (bottom panel). (b) On successful termination of all unorganized activity by a strong field shock, low-frequency (<10 Hz) point stimulation from the centre (white pulse sign) yielded slow conduction through the weakly coupled Kir2.1+Nav1.5 HEK-293 cells. Shown is a colour-coded map of cell activation, with white isochrone lines drawn at every 8 ms. Scale bar, 3 mm. (c) Following stable Cx43 overexpression, the derived Kir2.1+Nav1.5+Cx43 HEK-293 cells formed abundant intercellular Cx43 gap junctions (green), which were not detected in wt HEK-293 cells (inset). Scale bars, 10 μm. (d) Fluorescence recovery after photobleaching shows increased functional coupling in monoclonal Kir2.1+Nav1.5+Cx43 (Ex-293) cells (green squares;n=7) compared with wt HEK-293 (black diamonds;n=6) and Kir2.1+Nav1.5 HEK-293 (red triangles;n=5) cells. Palmitoleic acid (PA) inhibited junctional coupling and fluorescence recovery (blue circles;n=6). Error bars denote s.e.m. (e) Pacing in the centre of an Ex-293 monolayer elicited rapid and uniform AP spread (seeSupplementary Movie 1). Scale bar, 3 mm. Isochrones of cell activation (white lines) are labelled in milliseconds. Small black circles ina,b, andedenote 504 optical recording sites. DAPI, 4,6-diamidino-2-phenylindole. Figure 3: Stable overexpression of Cx43 in Kir2. 1+Na v 1.5 HEK-293 cells yields enhanced intercellular coupling and permits rapid AP propagation. ( a ) At the start of recording, confluent isotropic 2D networks (monolayers) of monoclonal Kir2.1+Na v 1.5 cells usually exhibited high-frequency unorganized electrical activity caused by numerous, slowly moving, splitting and colliding waves. Shown is one instant of optically recorded transmembrane voltage. Colour bar indicates percent AP amplitude (% APA). Different sites in the monolayer (for example, 1 and 2) activated at different rates (bottom panel), demonstrating the lack of spatial synchrony in activation. Red stars denote the time at which the transmembrane voltage frame (top panel) was taken. Scale bars indicate 3 mm (top panel) and 250 ms (bottom panel). ( b ) On successful termination of all unorganized activity by a strong field shock, low-frequency (<10 Hz) point stimulation from the centre (white pulse sign) yielded slow conduction through the weakly coupled Kir2.1+Na v 1.5 HEK-293 cells. Shown is a colour-coded map of cell activation, with white isochrone lines drawn at every 8 ms. Scale bar, 3 mm. ( c ) Following stable Cx43 overexpression, the derived Kir2.1+Na v 1.5+Cx43 HEK-293 cells formed abundant intercellular Cx43 gap junctions (green), which were not detected in wt HEK-293 cells (inset). Scale bars, 10 μm. ( d ) Fluorescence recovery after photobleaching shows increased functional coupling in monoclonal Kir2.1+Na v 1.5+Cx43 (Ex-293) cells (green squares; n =7) compared with wt HEK-293 (black diamonds; n =6) and Kir2.1+Na v 1.5 HEK-293 (red triangles; n =5) cells. Palmitoleic acid (PA) inhibited junctional coupling and fluorescence recovery (blue circles; n =6). Error bars denote s.e.m. ( e ) Pacing in the centre of an Ex-293 monolayer elicited rapid and uniform AP spread (see Supplementary Movie 1 ). Scale bar, 3 mm. Isochrones of cell activation (white lines) are labelled in milliseconds. Small black circles in a , b , and e denote 504 optical recording sites. DAPI, 4,6-diamidino-2-phenylindole. Full size image We derived 'Kir2.1+Na v 1.5+Cx43 HEK-293' monoclonal cell lines with bright mOrange fluorescence ( Fig. 1g ) and abundant expression of Cx43 gap junctions at cell–cell interfaces ( Fig. 3c ). One of these excitable and well-coupled Kir2.1+Na v 1.5+Cx43 HEK-293 monoclonal lines was named 'Excitable-293' (Ex-293). Functional intercellular coupling in Ex-293 cells was dramatically enhanced compared with endogenous HEK-293 coupling, as demonstrated by fluorescence recovery after photobleaching [27] , [29] ( Fig. 3d , Supplementary Fig. S3a,b and Supplementary Table S1 ) and dual whole-cell patch clamping [30] ( Supplementary Fig. S3c,d ). The average gap junctional conductance in Ex-293 cell pairs (134.1±14.0 nS (±s.e.m. ; n =12)) was comparable with that measured in isolated pairs of neonatal rat [28] or adult canine [31] cardiomyocytes. This Ex-293 monoclonal line, which has retained stable electrophysiological properties ( Supplementary Table S2 ) after multiple freeze–thaw cycles and more than 40 cell passages, was further utilized for the generation and characterization of biosynthetic excitable 2D and three-dimensional (3D) cell networks. When electrically stimulated, confluent 2D networks (monolayers) of randomly oriented Ex-293 cells supported rapid, spatially uniform AP propagation ( Fig. 3e , Supplementary Fig. S4a and Supplementary Movie 1 ) at excitation rates of up to 26.5 Hz and basic conduction velocities (CVs) of 23.3 cm s −1 . The dependence of CV in Ex-293 monolayers on the spatial distribution of gap junctions was explored by utilizing topographical and biochemical cues (microgrooved and micropatterned substrates [32] ) to elongate and align Ex-293 cells within confluent anisotropic networks and thin strands ( Supplementary Fig. S4b,c and Supplementary Movie 1 ). As expected, AP conduction was found to be faster along but slower across the aligned cells, as compared with non-aligned cells (longitudinal, transverse and isotropic velocity in Supplementary Table S2 ), due to the directional differences in the number of gap junctions (and cell–cell contacts) per unit length [3] . Expressed channels govern Ex-293 electrical function We further characterized how the expressed ion channels contribute to AP conduction in Ex-293 monolayers by using specific channel blockers. At the cellular level (assessed by sharp microelectrode recordings), gradual inhibition of I K1 by increasing doses of barium chloride (BaCl 2 ) significantly increased AP duration (APD 80 , Fig. 4a , Supplementary Fig. S5a ), depolarized RMP ( Fig. 4b ) and decreased the AP upstroke velocity ( Supplementary Fig. S5b ), confirming the important role of I K1 in AP repolarization, maintenance of RMP, and through the maintenance of the RMP, regulation of I Na availability and AP upstroke. Gradual inhibition of I Na by increasing doses of TTX, on the other hand, significantly decreased AP duration (APD 80 , Supplementary Fig. S5c ), upstroke velocity ( Fig. 4c and Supplementary Fig. S5d ) and amplitude ( Fig. 4d ) without a significant change in RMP (not shown), thereby confirming the prominent role of I Na in AP depolarization, and in conjunction with its opposing action on I K1 , regulation of AP duration. 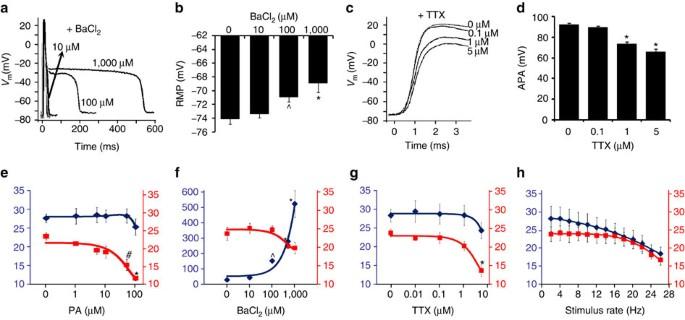Figure 4: Effects of channel blockers on the shape and conduction of APs in Ex-293 monolayers. (a–d) Dose-dependent effects ofIK1orINainhibition on the shape of propagated APs, recorded by sharp microelectrodes during 1-Hz stimulation. Inhibition ofIK1by increasing doses of BaCl2significantly prolonged AP duration (representative cell shown ina) and depolarized RMP (b;n=11–20). The rapid AP repolarization at high doses of BaCl2was likely contributed by the endogenous outward currents of HEK-293 cells (Supplementary Fig. S2). Inhibition ofINaby increasing doses of TTX decreased AP upstroke (representative cell shown inc) and amplitude (d;n=8–34). (e–g) Dose-dependent effects of specific channel blockers on CV (red squares) and AP duration (APD80, blue diamonds) in optically mapped Ex-293 monolayers during 1-Hz stimulation (n=5–7). Left (blue) and right (red) y axes correspond to APD80(ms) and CV (cm s−1), respectively. Highest doses shown are before conduction blocks occurred. (h) Effect of increased stimulation rate on CV (red squares) and APD80(blue diamonds). The rate was increased in 1-min steps, and data from all recording sites were averaged during the last 2 s of each step (n=5 monolayers). Error bars denote mean±s.e.m.; *P<0.001;#P<0.01; and ^P<0.05 vs corresponding drug-free values. Additional data for the effects of channel inhibition on AP shape and conduction are shown inSupplementary Figures S5andS6. Figure 4: Effects of channel blockers on the shape and conduction of APs in Ex-293 monolayers. ( a–d ) Dose-dependent effects of I K1 or I Na inhibition on the shape of propagated APs, recorded by sharp microelectrodes during 1-Hz stimulation. Inhibition of I K1 by increasing doses of BaCl 2 significantly prolonged AP duration (representative cell shown in a ) and depolarized RMP ( b ; n =11–20). The rapid AP repolarization at high doses of BaCl 2 was likely contributed by the endogenous outward currents of HEK-293 cells ( Supplementary Fig. S2 ). Inhibition of I Na by increasing doses of TTX decreased AP upstroke (representative cell shown in c ) and amplitude ( d ; n =8–34). ( e–g ) Dose-dependent effects of specific channel blockers on CV (red squares) and AP duration (APD 80 , blue diamonds) in optically mapped Ex-293 monolayers during 1-Hz stimulation ( n =5–7). Left (blue) and right (red) y axes correspond to APD 80 (ms) and CV (cm s −1 ), respectively. Highest doses shown are before conduction blocks occurred. ( h ) Effect of increased stimulation rate on CV (red squares) and APD 80 (blue diamonds). The rate was increased in 1-min steps, and data from all recording sites were averaged during the last 2 s of each step ( n =5 monolayers). Error bars denote mean±s.e.m. ; * P <0.001; # P <0.01; and ^ P <0.05 vs corresponding drug-free values. Additional data for the effects of channel inhibition on AP shape and conduction are shown in Supplementary Figures S5 and S6 . Full size image At the tissue level (assessed by macroscopic optical mapping of transmembrane potentials), inhibition of Kir2.1, Na v 1.5 or Cx43 channels by increasing doses of BaCl 2 , TTX or palmitoleic acid (PA), respectively, yielded gradual slowing of propagation ( Fig. 4e-g ) until conduction failure, thus demonstrating the critical roles of all the three expressed channels in AP conduction. Similarly, reduction of I Na by stimulation at progressively increasing rates [33] yielded a decrease in both CV and APD 80 ( Fig. 4h ). Furthermore, specific modulations of Na v 1.5 channel activity by lidocaine or flecainide [22] , [34] showed distinct effects on CV and APD 80 in Ex-293 monolayers during steady 10-Hz stimulation ( Supplementary Fig. S6a ). In addition to stimulated AP propagation, confluent Ex-293 monolayers supported self-sustained stationary (anchored to a small acellular obstacle, Fig. 5a–c ) or freely drifting ( Fig. 5d ) spiral waves ( Supplementary Movie 2 ), as is characteristic of various excitable media [35] including cardiac tissue [36] . The average rotational rates of single anchored and freely drifting spirals were 13.8±1.1 Hz (±s.e.m. ; n =5) and 18.8±1.6 Hz (±s.e.m. ; n =4), respectively. The application of BaCl 2 , PA or different inhibitors of I Na during the rotation of a stationary spiral wave slowed the rotation rate and eventually terminated all electrical activity in Ex-293 monolayers ( Fig. 5c and Supplementary Fig. S6b ). 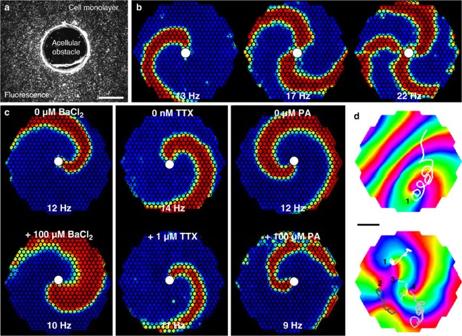Figure 5: Spiral waves in Ex-293 monolayers. (a) Coverslips with a 1.6-mm punched central hole were used to generate monolayers with an acellular obstacle. Scale bar, 1 mm. (b) Short bursts of rapid point stimulation (>25 Hz) from the monolayer periphery yielded formation of single or multiple spiral waves that anchored to the central obstacle (white circle) and rotated at shown rates. (c) Monolayers with a single stable anchored spiral were exposed to BaCl2, TTX or PA to decreaseIK1,INaor gap junctional coupling, respectively. The application of each blocker slowed spiral rotation, with BaCl2also causing an increase in AP duration (as evidenced by an increase in spiral wave width). Higher doses of the three compounds eventually terminated the spiral activity. Frames inbandcshow colour-coded optically recorded transmembrane voltage (blue to red denote rest to peak of AP), whereas small circles within these frames denote optical recording sites. (d) In the absence of a central obstacle, rapid stimulation occasionally caused the formation of single (top panel, shown in an anisotropic monolayer) or multiple (bottom panel shown in an isotropic monolayer) freely drifting spiral waves. Drift trajectories (overlay lines) of individual spiral tips (labelled by numbers) were tracked using phase map analysis and shown over a period of∼400 ms. The colours in the phase map denote different phases of the AP, with red colour showing the AP wave front. Scale bar, 4 mm. Representative movies of spiral waves are compiled inSupplementary Movie 2. Figure 5: Spiral waves in Ex-293 monolayers. ( a ) Coverslips with a 1.6-mm punched central hole were used to generate monolayers with an acellular obstacle. Scale bar, 1 mm. ( b ) Short bursts of rapid point stimulation (>25 Hz) from the monolayer periphery yielded formation of single or multiple spiral waves that anchored to the central obstacle (white circle) and rotated at shown rates. ( c ) Monolayers with a single stable anchored spiral were exposed to BaCl 2 , TTX or PA to decrease I K1 , I Na or gap junctional coupling, respectively. The application of each blocker slowed spiral rotation, with BaCl 2 also causing an increase in AP duration (as evidenced by an increase in spiral wave width). Higher doses of the three compounds eventually terminated the spiral activity. Frames in b and c show colour-coded optically recorded transmembrane voltage (blue to red denote rest to peak of AP), whereas small circles within these frames denote optical recording sites. ( d ) In the absence of a central obstacle, rapid stimulation occasionally caused the formation of single (top panel, shown in an anisotropic monolayer) or multiple (bottom panel shown in an isotropic monolayer) freely drifting spiral waves. Drift trajectories (overlay lines) of individual spiral tips (labelled by numbers) were tracked using phase map analysis and shown over a period of ∼ 400 ms. The colours in the phase map denote different phases of the AP, with red colour showing the AP wave front. Scale bar, 4 mm. Representative movies of spiral waves are compiled in Supplementary Movie 2 . Full size image Ex-293 cells form 3D biosynthetic excitable tissues To demonstrate our ability to generate de novo functional excitable tissues, we cultured Ex-293 cells within fibrin-based hydrogel constructs [37] . Using elastomeric molds and Velcro anchors, we created cm-sized 3D tissue cords ( Fig. 6a ). The Ex-293 cells in tissue cords compacted the hydrogel, aligned along the direction of passive tension imposed by the two Velcro anchors ( Fig. 6b,c ), and electrically coupled to form 3D-engineered tissues that supported uniform AP propagation ( Fig. 6d and Supplementary Movie 3 ), with an average CV and APD 80 of 18.1±1.7 cm s −1 and 33.5±1.2 ms, respectively (±s.e.m. ; n =7 tissue cords). 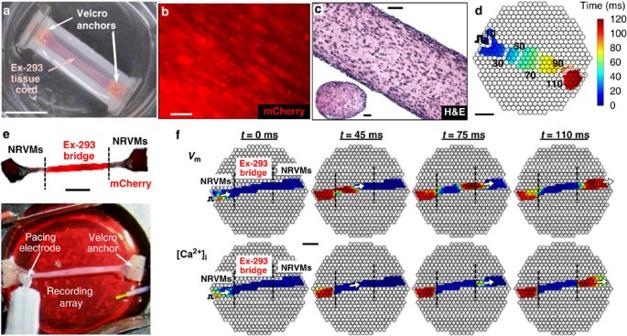Figure 6: Ex-293 cells form 3D biosynthetic excitable tissues and establish active electrical connection between remote regions in a 3D cardiac network. (a) A 3D tissue cord made by casting a mixture of Ex-293 cells and fibrin hydrogel within a tubular mold. Scale bar, 1 cm. (b) Longitudinal alignment of Ex-293 cells under passive tension inside a tissue cord. Scale bar, 50 μm. (c) Longitudinal and transverse histological sections of an Ex-293 tissue cord cultured for 4 weeks and stained with haematoxylin and eosin (H&E). Scale bars, 100 μm. (d) Point pacing at the periphery of an Ex-293 tissue cord (pulse sign) elicited rapid and uniform AP propagation (seeSupplementary Movie 3). Isochrones of cell activation (white lines) are labelled in milliseconds. Small black circles denote optical recording sites. Scale bar, 3 mm. (e) A cocultured-3D tissue cord with peripheral NRVM regions connected by a 1.3-cm-long central Ex-293 bridge (superimposed composite images of phase contrast and mCherry fluorescence). Scale bar, 5 mm. The optical recording array was placed underneath the cord (bottom panel). (f) Stimulation of a proximal NRVM region (left panel) generated a wave of transmembrane voltage (Vm) that spread (as shown by white arrow) through the Ex-293 tissue bridge and into the distal NRVM region (top frames). NRVM (but not Ex-293) excitation also yielded generation of intracellular calcium ([Ca2+]i) transients (bottom frames). Frames show colour-codedVmor [Ca2+]ioptically recorded at times shown above (blue to red indicate baseline to peak signal, respectively). Scale bar, 3 mm. Additional proof-of-concept examples where remote NRVM regions in 2D cultures are seamlessly connected by active AP propagation through Ex-293 cells are shown inSupplementary Figure S7andSupplementary Movie 4. Figure 6: Ex-293 cells form 3D biosynthetic excitable tissues and establish active electrical connection between remote regions in a 3D cardiac network. ( a ) A 3D tissue cord made by casting a mixture of Ex-293 cells and fibrin hydrogel within a tubular mold. Scale bar, 1 cm. ( b ) Longitudinal alignment of Ex-293 cells under passive tension inside a tissue cord. Scale bar, 50 μm. ( c ) Longitudinal and transverse histological sections of an Ex-293 tissue cord cultured for 4 weeks and stained with haematoxylin and eosin (H&E). Scale bars, 100 μm. ( d ) Point pacing at the periphery of an Ex-293 tissue cord (pulse sign) elicited rapid and uniform AP propagation (see Supplementary Movie 3 ). Isochrones of cell activation (white lines) are labelled in milliseconds. Small black circles denote optical recording sites. Scale bar, 3 mm. ( e ) A cocultured-3D tissue cord with peripheral NRVM regions connected by a 1.3-cm-long central Ex-293 bridge (superimposed composite images of phase contrast and mCherry fluorescence). Scale bar, 5 mm. The optical recording array was placed underneath the cord (bottom panel). ( f ) Stimulation of a proximal NRVM region (left panel) generated a wave of transmembrane voltage ( V m ) that spread (as shown by white arrow) through the Ex-293 tissue bridge and into the distal NRVM region (top frames). NRVM (but not Ex-293) excitation also yielded generation of intracellular calcium ([Ca 2+ ] i ) transients (bottom frames). Frames show colour-coded V m or [Ca 2+ ] i optically recorded at times shown above (blue to red indicate baseline to peak signal, respectively). Scale bar, 3 mm. Additional proof-of-concept examples where remote NRVM regions in 2D cultures are seamlessly connected by active AP propagation through Ex-293 cells are shown in Supplementary Figure S7 and Supplementary Movie 4 . Full size image Ex-293 cells restore active conduction in cardiac cultures We have previously demonstrated that unexcitable HEK-293 cells genetically engineered to express Cx43 can electrically couple with primary neonatal rat ventricular myocytes (NRVMs) [27] and passively connect them (with a long delay) over distances of up to a few hundred microns [32] . Ex-293 cells, on the other hand, both formed Cx43 gap junctions with NRVMs ( Supplementary Fig. S7a ) and, through fast active propagation, seamlessly connected remote (cm apart) cardiomyocyte regions in both 2D ( Supplementary Fig. S7b,c and Supplementary Movie 4 ) and 3D ( Fig. 6e,f ) NRVM networks. Thus, biosynthetic excitable cells and tissues could potentially act as actively conducting 'fillers' to restore fast and uniform AP propagation in diseased, slow-conducting excitable tissues. This study introduces a methodology for the de novo generation of actively conducting excitable tissues from unexcitable somatic cells by the stable forced expression of only three membrane channels. Specifically, through a stepwise experimental approach ( Fig. 1 and Supplementary Fig. S1 ), we showed that genetic engineering of: significant membrane polarization by introduction of Kir2.1 channels; rapid depolarization capacity by introduction of Na v 1.5 channels; and robust intercellular coupling by overexpression of Cx43 gap junctions synergistically enabled electrical excitability and conduction in HEK-293 cells. Previously, Hsu et al . [38] transiently expressed voltage-gated sodium (Na v 1.2) and potassium (Shaker H4) channels in CHO cells, but because the average RMP of these cells was −26.8 mV, APs could be induced only under electronically applied current-clamp hyperpolarization. More recently, Cho et al . [39] have transiently expressed the Kir2.1 channel and a slow bacterial sodium channel (NaChBac) in HEK-293 cells to yield slow rising and long APs in 5/31 cells, whereas Abraham et al . [40] have expressed Cx43 to promote electrical coupling of skeletal myotubes and decrease their arrhythmogenic effects in cocultures with cardiomyocytes. We, on the other hand, have created stable excitable cell lines with reproducible electrical properties including fast rising (dV/dt max ≈150 V s −1 ) and rapidly propagating (CV≈23 cm s −1 ) APs. As these cells can be assembled into autonomous, actively conducting tissues, we were able to pharmacologically dissect the specific roles of each expressed channel in the dynamics of AP conduction and demonstrate the ability of these biosynthetic tissues to restore fast conduction within arbitrary size gaps in cardiomyocyte cultures. Single unexcitable cells have been traditionally used in heterologous expression systems in conjunction with patch-clamp recordings to isolate and study the function of specific ion channels [41] . The biosynthetic excitable cells described in this study can be additionally utilized as a tissue–scale heterologous expression system to directly investigate not only specific channel activity in single cells but also AP conduction in multicellular networks fabricated from these same cells. For example, in this study, we have isolated and quantified the role of Na v 1.5 in AP generation and conduction during control conditions as well as different pharmacological challenges in both single cells and cell networks. In general, biosynthetic excitable tissues as a well-defined, reproducible and versatile platform could complement studies in primary excitable cells by helping elucidate the distinct roles that specific ion channels and gap junctions, their mutations [42] , [43] , [44] , [45] auxiliary subunits [46] , or accessory proteins [47] , [48] have in tissue-level electrophysiology. Furthermore, the potential to efficiently manipulate the gene expression and spatial organization of engineered cells within biosynthetic tissues can allow for well-controlled experiments to validate and advance existing theoretical and computational models of AP conduction as well as facilitate the design of robust and reproducible cell-based biosensors [49] . Importantly, we also performed proof-of-concept in vitro studies showing that biosynthetic excitable cells and tissues can establish a fast and seamless electrical connection between distant cardiomyocytes. The implantation of stem cells or somatic cells with genetically engineered electrical properties has been proposed as a potential strategy to improve compromised electrical function in the heart [50] , [51] , [52] , [53] . For example, unexcitable cells with engineered potassium channels have been applied to locally modify cardiac conduction through coupling with cardiomyocytes [54] . However, because of their unexcitable nature, these cells would still fail to propagate over distances larger than a few hundred microns [32] , [55] . In contrast, the use of autonomously conducting biosynthetic cells with basic electrical properties tailored to mimic those of the host tissue could allow functional repair of arbitrary size conduction defects. For example, slow tortuous conduction at the site of myocardial infarct [56] could be enhanced by implanting biosynthetic excitable cells or genetically modifying endogenous fibroblasts to establish direct paths of fast AP propagation. For potential clinical use, however, highly proliferative HEK-293 cells would have to be replaced by another contact-inhibited, terminally differentiated and readily accessible cell source. Overall, we believe that our approach not only opens the door to novel studies of electrical conduction but also, through further integration of electrophysiology, synthetic biology and tissue engineering, the development of new treatments for excitable tissue disorders. Cloning of rat connexin-43 gene ( GJA1 ) Total RNA was extracted and purified from isolated NRVMs (Qiagen, RNeasy Kit). Reverse transcription with oligo(dT) primers was performed to synthesize first-strand complementary DNA (Bioline, cDNA Synthesis Kit). The cDNA was used as the template in a standard PCR reaction. PCR primers were designed based upon the published coding sequence for rat connexin-43 (GenBank no. NM_012567). The amplified PCR product was verified by nucleotide sequencing and subcloned into the pCMV5(CuO)–IRES–mOrange expression plasmid. Generation of engineered cell lines The human KCNJ2 , SCN5A and rat GJA1 cDNAs were subcloned into a bicistronic expression vector (pCMV5(CuO)–IRES–GFP, Qbiogene). The genes encoding mCherry and mOrange [18] were used to replace GFP in the KCNJ2 and GJA1 plasmids, respectively. HEK-293 cells (ATCC, CRL-1573) were cultured, transfected and selected for stable expression using previously described methods [27] . The Ex-293 line was established by three successive single-plasmid (Kir2.1, Na v 1.5 and then Cx43) transfections, with monoclonal isolation and expression analysis before each transfection. Whole-cell membrane current recordings HEK-293 cells were gently trypsinized and plated onto clean glass coverslips for recording. Patch electrodes were fabricated with tip resistances of 0.8–1.8 MΩ (for I Na ) or 1.5–3.5 MΩ (for I K1 , AP, current or dual clamp) when filled with internal patch solutions. Whole-cell currents were recorded at room temperature using the Multiclamp 700B amplifier (Axon Instruments), filtered with a 10-kHz Bessel filter, digitized at 40 kHz and stored on a computer. Data was acquired and analyzed using WinWCP software (John Dempster, University of Strathclyde). The internal and external solutions and voltage-clamp protocols for recording of I Na and I K1 were similar to other published studies [33] , [57] . Whole-cell membrane voltage and AP voltage-clamp recordings Cell intracellular potential was recorded at room temperature in current-clamp mode (no holding current) in response to 1-ms depolarizing current steps (from 0.5 nA to 2 nA in 0.1-nA increments) in an attempt to elicit an all-or-none AP response. Extracellular bath solution (Tyrode's) consisted of (mM) 135 NaC1, 5.4 KCl, 1.8 CaCl 2 , 1.0 MgCl 2 , 0.33 NaH 2 PO 4 , 5 HEPES and 5 glucose (pH 7.4). The membrane current during the course of AP was accessed using the AP-clamp technique [24] , in which a previously recorded AP waveform (measured in an excitable Ex-293 monolayer at 35 °C with a sharp electrode) was used as the stimulus protocol in whole-cell voltage-clamp mode. Recorded currents in the presence of 1 mM BaCl 2 or 5 μM TTX reflected respective contributions of I Na and I K1 to the AP waveform. Dual whole-cell patch-clamp recordings HEK-293 cell pairs that were formed in sparsely plated 2-day cultures were used for dual whole-cell measurement of gap junctional conductance, as previously described [30] . Patch electrodes (1.5–3.5 MΩ resistance) were filled with a CsCl-containing solution to block endogenous potassium currents. Each cell in the pair was clamped by a separate patch electrode to a 0-mV holding potential. A 20-mV depolarizing (8-s long) pulse was then applied to one of the two cells. Gap junctional conductance ( G j ) was then calculated by dividing the resulting junctional current by the transjunctional voltage step (+20 mV) after accounting for the uncompensated series resistance in each electrode [58] . Sharp intracellular recordings HEK-293 monolayers were placed into a temperature-controlled (35 °C) chamber mounted onto an inverted microscope (Nikon, Eclipse TE2000), perfused with warm Tyrode's solution and stimulated at 1 Hz by a bipolar point electrode connected to a Grass Stimulator (Grass Technologies). Propagated APs were recorded 6 mm away from the stimulus site using a sharp intracellular electrode (50–80 MΩ tip resistance), as previously described [27] . Data was low-pass filtered through a 4.5-kHz Butterworth filter, sampled at 20 kHz using a Multiclamp 700B amplifier (Axon Instruments) and recorded using WinWCP or Chart software. RMP, AP amplitude, duration at 80% repolarization (APD 80 ) and maximum upstroke velocity (dV m dt −1 ) were measured using a custom-made MATLAB program [59] . Fluorescence recovery after photobleaching Functional coupling in HEK-293 cells was assessed using fluorescence recovery after photobleaching [29] , as described previously [27] . HEK-293 monolayers were loaded with Calcein AM dye (Molecular Probes, 0.5 μM, 20 min at 37 °C) and washed in phosphate-buffered saline. The target cell was photobleached with a 488-nm Argon laser and imaged every 10 s for the following 6 min using an upright confocal microscope (Zeiss, LSM 510). The time course of recovery of calcein fluorescence in the target cell (by inflow from the adjacent cells) was fit by an exponential curve using custom-made MATLAB software. The calculated recovery rate constant [29] for each sample was normalized by the number of cells in direct contact with the target cell. Fabrication of excitable 2D HEK-293 networks Isotropic excitable HEK-293 (Ex-293) monolayers were made by plating 2.5×10 5 cells onto fibronectin-coated (15 μg ml −1 , Sigma) Aclar (Electron Microscopy Sciences) coverslips (22-mm diameter) and culturing to confluence. Anisotropic Ex-293 monolayers and thin strands were made by culturing cells on fibronectin-coated microgrooved films (Edmund Industrial Optics) or microcontact-printed fibronectin lines [32] , respectively. Fabrication of 3D tissue constructs Fibrin-based hydrogel solution was made using bovine fibrinogen (2 mg ml −1 , Sigma), bovine thrombin (0.4 U mg −1 fibrinogen, Sigma) and Matrigel (10% v/v, Becton Dickinson), as previously described [37] . The 3D tissue cords were fabricated by casting 7×10 6 cells per ml hydrogel solution inside a 2.5-cm-long silicon half-tube with two Velcro felts (3M Company; St Paul, MN) pinned at the tube ends. The Velcro anchored the hydrogel and, by establishing passive tension during cell-mediated gel compaction, facilitated cell spreading and contact. Aminocaproic acid (1 mg ml −1 , Sigma) was added to the culture medium to prevent degradation of fibrin by serum plasmin. To create an NRVM tissue cord with a central Ex-293 bridge, three tips of a multichannel pipette were used to simultaneously inject Ex-293/hydrogel solution in the middle and NRVM/hydrogel solutions at the two ends of the silicon half-tube. With time in culture, NRVMs and Ex-293 cells spread, aligned and coupled while maintaining distinct spatial boundaries, as identified by fluorescence imaging for GFP, mCherry and mOrange. Optical mapping of impulse propagation The 2D cell networks and 3D tissue constructs were stained with a voltage-sensitive dye, Di-4 ANEPPS (10 μM, 5–7 min), or a non-ratiometric Ca 2+ -sensitive dye, X-Rhod-1 (3 μM, 45 min). Transmembrane voltage and intracellular Ca 2+ concentration, [Ca 2+ ] i , were optically mapped with 504 optical fibres arranged into a 20-mm diameter hexagonal bundle (Redshirt Imaging), as previously described [32] , [59] . Fluorescence signals were converted to voltage by photodiodes and acquired at a 2.4-kHz sampling rate with macroscopic (750 μm) or microscopic (37.5 μm, ×20 magnification) spatial resolution. To prevent motion artefacts, cells were exposed to 10-μM blebbistatin (Sigma). An XYZ-micropositioned platinum point electrode was used to initiate electrical conduction at progressively higher pacing rates (1–30 Hz in 30-s steps) [60] . Data were processed, displayed and analyzed using custom-made MATLAB software. The longitudinal and transverse CV, velocity anisotropy ratio, APD 80 , maximum capture rate (where each stimulus was still followed by an AP response) and CV and APD 80 rate dependence curves were derived, as previously described [59] , [60] . Studies of spiral activity Spiral waves were induced by rapid (25–30 Hz) burst pacing from the edge of a cell monolayer and optically mapped [60] . For anchored (anatomical) spiral wave studies, a 1.6-mm circular obstacle was punched out from the centre of a coverslip before cell seeding. Spiral rotational rate was calculated by averaging activation rate from multiple sites at the coverslip periphery. Phase map and singularity analyses (with 15-ms time delay) were used to track the tip trajectory of drifting spiral waves [25] , [60] . During perfusion of channel inhibitors, rotational rate, wave unpinning and changes in spiral wave path length were documented until termination of reentrant activity. Pharmacological studies TTX (Sigma), BaCl 2 (Alfa Aesar) and PA (Sigma) were added to extracellular bath solution during patch clamping or optical mapping (1 Hz, 1.2× threshold stimulation in monolayers) recordings to selectively inhibit I Na , I K1 and gap junctional coupling, respectively. Recordings with lidocaine (50 μM, Sigma) or flecainide (10 μM, Sigma) were performed during 40 pulses at 10-Hz stimulation. All recordings using pharmacological modulation were started 5 min after drug application. Immunostaining Cells were immunostained, as previously described [27] . Anti-sarcomeric α-actinin (Sigma, EA-53 mouse monoclonal) and anti-connexin-43 (Zymed, rabbit polyclonal) primary antibodies were applied overnight at 4 °C. Secondary Alexa Fluor 488 (chicken anti-rabbit) and Alexa Fluor 594 (chicken anti-mouse) antibodies were applied for 1 h at room temperature. Nuclei were counterstained with DAPI (Sigma). All fluorescent images were acquired, pseudocoloured and processed using IPLab (BioVision Technologies), as previously described [27] . Tissue bundles were fixed in 4% PFA overnight, paraffin embedded, cut into 5-μm-thick transverse and longitudinal sections, stained with haematoxylin & eosin (Duke Pathology Department) and imaged using an inverted microscope (Nikon, TE2000) and NIS-Elements software (Nikon). Statistical analysis Data are presented as mean±s.e.m. and were evaluated for statistical significance using linear regression or an analysis of variance (one-way, α-factor of 0.05), followed by Tukey's post hoc test for multiple comparisons. Statistical significance was defined as ^ P <0.05, # P <0.01 and * P <0.001. How to cite this article : Kirkton, R. D. and Bursac, N. Engineering biosynthetic excitable tissues from unexcitable cells for electrophysiological and cell therapy studies. Nat. Commun. 2:300 doi: 10.1038/ncomms1302 (2011).